Intramuscular adipogenesis is inhibited by myo-endothelial progenitors with functioning Bmpr1a signalling Developing human muscle contains inter-myofibre progenitors expressing Bmp-receptor 1a (Bmpr1a) and Myf5 that respond to stimulation with Bmp4. Here we ablate Bmpr1a in Myf5- and MyoD-expressing cells in vivo . Mutant mice reveal increased intramuscular fat and reduced myofibre size in selected muscles, or following muscle injury. Myo-endothelial progenitors are the most affected cell type: clonal studies demonstrate that ablation of Bmpr1a in myo-endothelial cells results in decreased myogenic activity, while adipogenic differentiation is significantly increased. Downstream phospho-Smad 1, 5, 8 signalling is also severely decreased in mutant myo-endothelial cells. Lineage tracing of endothelial cells using VE-cadherin Cre driver failed to reveal a significant contribution of these cells to developing or injured skeletal muscle. Thus, myo-endothelial progenitors with functioning Bmpr1a signalling demonstrate myogenic potential, but their main function in vivo is to inhibit intramuscular adipogenesis, both through a cell-autonomous and a cell–cell interaction mechanism. Skeletal muscle exhibits sustained regenerative capacity in response to acute injury or disease. This remarkable regenerative capacity is thought to be largely due to satellite cells, the tissue-specific stem cells located beneath the basal lamina of mature myofibres [1] , [2] , [3] . Quiescent satellite cells in adult muscle express the transcription factor Pax7, while their activation is marked by co-expression of Myf5 and MyoD [4] , [5] , [6] , [7] . Myf5 and MyoD can partially compensate for one another during development [8] , [9] , [10] , although they also have distinct functions [11] . Besides satellite cells, other progenitors with myogenic activity have been identified [12] . This heterogeneous group includes cells located interstitially between muscle fibres or tightly associated with the capillaries [13] , [14] , [15] , [16] , [17] . Despite accumulating evidence that inter-myofibre cells that do not express myogenic markers can adopt a myogenic fate [16] , [18] , their function in postnatal muscle remains poorly understood. Studies have indicated that during myogenic regeneration inter-cellular interactions occur between myogenic and fibro-adipogenic cells [19] , [20] , [21] , [22] , but the exact signals that regulate this process have not been elucidated. In addition, multipotential interstitial progenitors within skeletal muscle hypersensitive to Bmp signalling are likely responsible for heterotopic ossification observed in fibrodysplasia ossificans progressiva (FOP), but these cells do not derive from the endothelium [23] . Our previous studies in human fetal skeletal muscle concluded that Bmp signalling is important for the proliferation of interstitial progenitors, which co-express Myf5 and Bmpr1a [24] . However, neither the myogenic differentiation potential of these progenitors in developing or adult muscle nor the consequences of altering Bmpr1a signalling in vivo are known. In the present study, we ablated Bmpr1a signalling in cells expressing the myogenic markers Myf5 or MyoD . Myf5 +/Cre :Bmpr1a f/f mice were born runted and remained small throughout life, with several epaxial muscles (paraspinal, neck and trapezius) exhibiting severely decreased size, accompanied by increased intramuscular fat. Limb muscle injury with cardiotoxin (CTX) also led to significant accumulation of fat tissue in mutant mice of both genotypes. Analyses of wild-type and mutant muscles revealed that a subfraction of endothelial cells (Sca-1 pos CD45 neg CD31 pos PDGFRα neg , named MECs) exhibits myogenic potential and suppresses the differentiation of intramuscular adipocytes when Bmpr1a signalling is unaffected. When Bmpr1a signalling is disrupted, MEC cells lose their myogenic differentiation potential and instead exhibit increased adipogenic potential. In addition, their ability to suppress intramuscular adipocytes is severely inhibited. Thus, myo-endothelial progenitors with functioning Bmpr1a signalling adopt a myogenic fate and act as suppressors of intramuscular fat formation. Bmp signalling in this subfraction of endothelial cells could act as a key regulator for balance between muscle and fat. Conditional ablation of Bmpr1a in Myf5 and MyoD progenitors To study the role of Bmpr1a signalling in myogenic cells, Bmpr1a f/f mice [25] were crossed with mice expressing Cre under the control of the Myf5 promoter ( Myf5 +/Cre ) [26] . Myf5 +/Cre :Bmpr1a f/f mice were born runted and remained significantly smaller than wild-type (WT) littermates throughout life ( Fig. 1a ). The body weight of Myf5 +/Cre :Bmpr1a f/f conditional knockout (KO) mice was significantly reduced compared with WT littermates ( Fig. 1b ). Gross examination revealed that the dorsal skeletal muscles from KO mice were smaller than that in WT mice ( Fig. 1c ). Normalization of the individual muscle weight to the total body weight confirmed significant difference in size of the mutant epaxial muscles, including the paraspinal and trapezius ( Fig. 1d ). To examine whether the myofibre number and/or size was altered in conditionally ablated Bmpr1a mutant muscles, cross-sections of paraspinal and trapezius muscles from WT and KO animals were compared at the same anatomical position to ensure that any difference observed was not due to the plane of sectioning. The transverse area of the entire paraspinal muscle bundle was notably smaller in Myf5 +/Cre :Bmpr1a f/f mice than in WT mice ( Fig. 1e ), with a significantly lower number of myofibres in Myf5 +/Cre :Bmpr1a f/f muscles ( Fig. 1f ). Reduced myofibre size was observed in both paraspinal and trapezius mutant muscles ( Fig. 1h,j ), accompanied by fat accumulation ( Fig. 1g,i , yellow arrows), which was confirmed by Oil red O staining ( Supplementary Fig. 1A ) and by the increased expression of the adipocyte marker fatty acid synthase (Fasn, Supplementary Fig. 1D ). In contrast, the tibialis anterior (TA) and gastrocnemius (GA) muscles did not reveal significant differences in myofibre size ( Supplementary Fig. 1E,F,H,I,K ). Since Myf5 pos myogenic progenitors contribute mostly to epaxial muscles, such as paraspinal, intercostal and trapezius [27] , while MyoD pos progenitors contribute to hypaxial muscles, including limb muscles [28] , we asked whether Bmpr1a function might be linked to both myogenic cell lineages. A second knockout mouse model was generated by crossing MyoD +/iCre (ref. 29 ) to Bmpr1a f/f mice. MyoD +/iCre :Bmpr1a f/f mice had the same body weight as control mice and the hypaxial muscles (TA and GA) revealed no significant differences compared with controls both histologically and in myofibre cross-sectional area ( Supplementary Fig. 1G,J,K ). The paraspinal muscle also appeared unaffected in MyoD +/iCre :Bmpr1a f/f mice ( Supplementary Fig. 1C ). Bmpr1a expression was analysed via quantitative RT-PCR using 5–6 animals per cohort, and it was significantly reduced in nearly all Myf5 +/Cre :Bmpr1a f/f skeletal muscles examined, except for the diaphragm ( Supplementary Fig. 1M ), suggesting that development of the diaphragm muscle might differ from other skeletal muscles, which is not surprising given its complex anatomical structure [30] . Similarly, expression of Bmpr1a mRNA was significantly decreased in muscles from MyoD +/iCre :Bmpr1a f/f mice ( Supplementary Fig. 1N ). Thus, while expression of Bmpr1a was effectively reduced in both Myf5 and MyoD progenitors, Myf5 +/Cre :Bmpr1a f/f mice exhibited more obvious abnormalities, suggesting that Bmpr1a function might be more prominent in Myf5 progenitors. 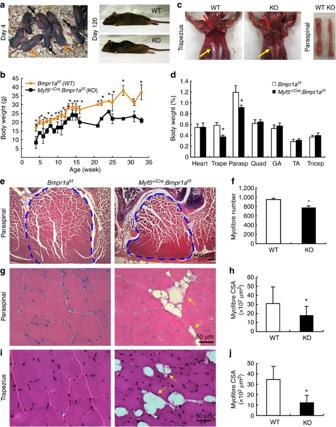Figure 1:Myf5+/Cre:Bmpr1af/fmice are born runted with small epaxial muscles. (a,b) Body size and weight ofMyf5+/Cre:Bmpr1af/f(KO) mice compared withBmpr1af/f(WT) littermates. Adult KO mice exhibit severe kyphosis, indicating the weakness of the dorsal muscles. Black arrows point to KO mice, orange arrows to WT littermates. (b) Body weight comparison was derived from female mice and data are presented as mean±s.d. byt-test (n=6; *P<0.05). Similar results were seen with male mice (Supplementary Fig. 1L). (c) Trapezius (red arrow) and paraspinal (yellow arrow) muscles in WT and KO littermate mice. (d) Normalization of tissue masses with total body weight (n=3; *P<0.05). Trape: trapezius; Parasp: paraspinal; GA: gastrocnemius; TA: tibialis anterior. (e) H&E staining of transverse sections of paraspinal muscle bundle (outlined by the blue dotted line) inBmpr1af/f(WT) andMyf5+/Cre:Bmpr1af/fmice (mean±s.d. 53,320±5,756 μm2KO versus 102,977±16,416 μm2for WT,P<0.05). (f) A significant reduction in the number of myofibres was observed in mutant animals (mean±s.d. 784±52 inMyf5+/Cre:Bmpr1af/fversus 949±48 in WT,t-test *P<0.05,n=3). (g,i) Presence of adipocytes (yellow arrows) and (h,j) reduced cross-sectional area (CSA) were also seen in mutant paraspinal and trapezius muscles, respectively (n=3; *P<0.05). Error bars in (f,h,j) represent the s.d. Figure 1: Myf5 +/Cre :Bmpr1a f/f mice are born runted with small epaxial muscles. ( a , b ) Body size and weight of Myf5 +/Cre :Bmpr1a f/f (KO) mice compared with Bmpr1a f/f (WT) littermates. Adult KO mice exhibit severe kyphosis, indicating the weakness of the dorsal muscles. Black arrows point to KO mice, orange arrows to WT littermates. ( b ) Body weight comparison was derived from female mice and data are presented as mean±s.d. by t -test ( n =6; * P <0.05). Similar results were seen with male mice ( Supplementary Fig. 1L ). ( c ) Trapezius (red arrow) and paraspinal (yellow arrow) muscles in WT and KO littermate mice. ( d ) Normalization of tissue masses with total body weight ( n =3; * P <0.05). Trape: trapezius; Parasp: paraspinal; GA: gastrocnemius; TA: tibialis anterior. ( e ) H&E staining of transverse sections of paraspinal muscle bundle (outlined by the blue dotted line) in Bmpr1a f/f (WT) and Myf5 +/Cre :Bmpr1a f/f mice (mean±s.d. 53,320±5,756 μm 2 KO versus 102,977±16,416 μm 2 for WT, P <0.05). ( f ) A significant reduction in the number of myofibres was observed in mutant animals (mean±s.d. 784±52 in Myf5 +/Cre :Bmpr1a f/f versus 949±48 in WT, t -test * P <0.05, n =3). ( g , i ) Presence of adipocytes (yellow arrows) and ( h , j ) reduced cross-sectional area (CSA) were also seen in mutant paraspinal and trapezius muscles, respectively ( n =3; * P <0.05). Error bars in ( f , h , j ) represent the s.d. Full size image Muscle regeneration in mutant mice leads to increased fat Bmpr1a mRNA is transiently upregulated from day 3 to day 5 post-cardiotoxin (CTX) injury in WT mice ( Fig. 2a ), a time when myogenic progenitors are activated for repair [31] , [32] . The muscle regenerative capacity of Bmpr1a f/f (control), Myf5 +/Cre :Bmpr1a f/f and MyoD +/iCre :Bmpr1a f/f mice were assayed in parallel. After 7 days, centrally nucleated myofibres were seen in all genotypes, indicating ongoing regeneration; however, mutant mice displayed increased fat infiltration, as confirmed by Oil Red O staining ( Fig. 2b ). The mRNA levels of the adipogenic transcription factor peroxisome proliferator-activated receptor γ (PPARγ) and the fatty acid-binding protein 4 (FABP4, also known as aP2) were significantly elevated in injured mutant muscle ( Fig. 2c ). In addition, regenerated myofibres were significantly smaller in Myf5 +/Cre :Bmpr1a f/f and MyoD +/iCre :Bmpr1a f/f mice compared with controls by t -test ( P <0.05) ( Fig. 2d ). At day 18 after CTX injection, mutant muscles still exhibited a significant amount of fat accumulation, and the diameter of regenerated myofibres was 15% smaller in Myf5 +/Cre :Bmpr1a f/f mice compared with controls ( P <0.01) ( Fig. 2e ). Similar results were seen in injured GA muscle. Recent studies have reported that TGFβ signalling can affect myofibre size through ALK4 and ALK5 type I activin receptors (which signal via pSmad 2,4) [33] . In addition, Bmp signalling through pSmad 1,5,8 can affect myofibres size via downstream signalling through mTOR [34] . Given that Bmpr1a is known to signal via pSmad 1,5,8 (ref. 35 ), we examined phosphorylation of Smad1/5/8 and Smad2 in uninjured and injured muscles from WT and Myf5 +/Cre :Bmpr1a f/f (KO) mice ( Supplementary Fig. 2A ). Phospho-smad1/5/8 levels were slightly reduced in epaxial muscles as well as in cardiotoxin-injured TA muscles from KO mice. In contrast, pSmad2 expression was similar between WT and KO muscles, suggesting ablation of Bmpr1a does not affect signalling through pSmad2. 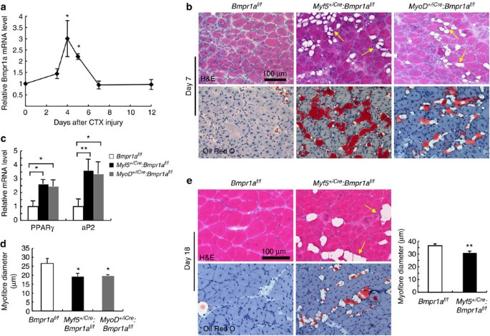Figure 2: Increased fat infiltration and decreased myofibre size in regenerating mutant muscle. (a) Transient upregulation of Bmpr1a mRNA in regenerating TA muscle of WT mice following CTX injury. Results are shown as mean±s.d. (n=3, *P<0.05). (b) H&E staining of cross-sections of TA muscles 7 days after CTX injury. Lipid accumulation in mutant mice (yellow arrows) was confirmed by Oil Red O staining. (c) Expression of the adipogenic transcription factor PPARγ and the mature adipocyte marker aP2 were assessed by real-time qRT-PCR 4 days post-injury. Both were significantly increased in regenerating muscle from mutant mice (n=3–4; *P<0.05; **P<0.01. Error bars define the s.d. value). (d) Average myofibre diameter was significantly greater in regenerating TA muscle of controlBmpr1af/fmice (26.6±2.8 μm) compared withMyf5+/Cre:Bmpr1af/f(19.3±1.8 μm) andMyoD+/Cre:Bmpr1af/fmice (19.7±0.6 μm) 7 days following CTX injury. Data were averaged (n=4 mice/group) and expressed as mean±s.d. (*P<0.05). (e) H&E (upper panels) and oil-red O staining (lower panels) of regenerating WT and KO tibialis anterior (TA) muscle 18 days following CTX injury. Fat accumulation (indicated by arrows) is still observed, as is a significantly reduced myofibre size in mutant mice (30.9±1.3 μm versus 36.5±1.4 μm for control) (n=3, **P<0.01). Figure 2: Increased fat infiltration and decreased myofibre size in regenerating mutant muscle. ( a ) Transient upregulation of Bmpr1a mRNA in regenerating TA muscle of WT mice following CTX injury. Results are shown as mean±s.d. ( n =3, * P <0.05). ( b ) H&E staining of cross-sections of TA muscles 7 days after CTX injury. Lipid accumulation in mutant mice (yellow arrows) was confirmed by Oil Red O staining. ( c ) Expression of the adipogenic transcription factor PPARγ and the mature adipocyte marker aP2 were assessed by real-time qRT-PCR 4 days post-injury. Both were significantly increased in regenerating muscle from mutant mice ( n =3–4; * P <0.05; ** P <0.01. Error bars define the s.d. value). ( d ) Average myofibre diameter was significantly greater in regenerating TA muscle of control Bmpr1a f/f mice (26.6±2.8 μm) compared with Myf5 +/Cre :Bmpr1a f/f (19.3±1.8 μm) and MyoD +/Cre :Bmpr1a f/f mice (19.7±0.6 μm) 7 days following CTX injury. Data were averaged ( n =4 mice/group) and expressed as mean±s.d. (* P <0.05). ( e ) H&E (upper panels) and oil-red O staining (lower panels) of regenerating WT and KO tibialis anterior (TA) muscle 18 days following CTX injury. Fat accumulation (indicated by arrows) is still observed, as is a significantly reduced myofibre size in mutant mice (30.9±1.3 μm versus 36.5±1.4 μm for control) ( n =3, ** P <0.01). Full size image To determine whether the reduced regenerative capacity of Myf5 +/Cre :Bmpr1a f/f muscle was due to a decreased number of satellite cells, the number of Pax7 pos cells was assessed by immunohistochemistry on cross-sections of TA muscles either uninjured or 7 days post CTX injury ( Supplementary Fig. 2B , arrows). No significant differences in the number of Pax7 pos cells were seen between the genotypes ( Supplementary Fig. 2C ). To confirm these results, Pax7 expression was examined via quantitative real-time RT-PCR and western blot ( Supplementary Fig. 2D ). Again, no significant differences were observed between control and mutant mice in either uninjured or regenerating muscle. Mutant myo-endothelial cells lose myogenic potential To identify the cell type(s) responsible for the increased fat accumulation in mutant muscle, multiple cell fractions, including satellite cells (SCs); endothelial and myo-endothelial cells (MECs); and adipogenic progenitors (APs), were isolated by FACS as outlined in Supplementary Fig. 3 . Satellite cells were isolated as Sca-1 neg CD45 neg CD31 neg CD106 pos cell fraction ( Supplementary Fig. 3G ), as previously described [36] , [37] . Endothelial and myo-endothelial cells were isolated as Sca-1 pos CD45 neg CD31 pos PDGFRα neg cells ( Supplementary Fig. 3H ). Adipogenic progenitors were purified as Sca-1 pos CD45 neg CD31 neg cells, which were also >95%PDGFRα pos ( Supplementary Fig. 3F,I ). To validate the purity of freshly isolated SCs, MECs and APs, the purified cell fractions were assessed for expression of Sca-1 and CD31 following cytospin ( Supplementary Fig. 4 ). As expected, all MECs were Sca-1 pos CD31 pos , SCs were Sca-1 neg CD31 neg , while APs were Sca-1 pos CD31 neg , suggesting minimal or no overlap among these cell groups. Given the possibility that MECs could overlap with other cell fractions previously described, such as mesoangioblasts and pericytes [38] , [14] , [17] , PICs [16] , [39] , [40] and beta-4 integrin pos (β4-ITG) interstitial myogenic progenitors [41] , expression of additional markers was tested in MECs, APs and SCs ( Supplementary Fig. 5 ). By FACS analysis, a small fraction of MECs expressed β4-ITG (~10%, Supplementary Fig. 5A ), while by qRT/PCR MECs expressed PDGFRβ, NG2 and PW1 at lower levels as compared with APs and SCs ( Supplementary Fig. 5B ). Semi-quantitative RT/PCR followed by gel separation of the PCR products confirmed the presence of PDGFRβ expression in MECs, while no bands were seen following amplification of NG2 or PW1 mRNAs in MECs ( Supplementary Fig. 5C ). Of note, SCs expressed PW1 mRNA, a result in agreement with previously published data [40] . These results were confirmed by antibody staining on cytospins of freshly isolated MECs. Within a total 500–700 MECs analysed, 5.3% were positive for PDGFRβ, 0.6% were positive for NG2 and 0.5% were positive for smooth muscle actin (SMA) ( Supplementary Fig. 5D,E ). To study the in vitro differentiation potential of SCs, MECs and APs, the cell fractions were isolated in parallel from control and Myf5 +/Cre :Bmpr1a f/f mice and cultured in conditions that favour myogenic or adipogenic differentiation ( Fig. 3 ). SCs isolated from WT and mutant mice differentiated robustly into myotubes, under either myogenic ( Fig. 3a,b ) or adipogenic differentiation condition ( Supplementary Fig. 6A ), with no differences detected between the genotypes despite the fact that Bmpr1a expression was severely decreased in mutant SCs and MECs ( Fig. 3e ). MECs are a mixed population containing both endothelial and myo-endothelial cells, and a subfraction of MECs attach to the tissue culture plates when cultured. These cultured MECs from WT mice differentiated consistently into myotubes, regardless of whether they were cultured in myogenic ( Fig. 3c ) or adipogenic differentiation conditions ( Fig. 3f ), suggesting MECs can adopt a myogenic fate in vitro. In contrast, MECs from mutant mice with severely reduced Bmpr1a expression showed decreased myogenic differentiation potential ( Fig. 3d ) and presence of mature adipocytes when differentiated in adipogenic medium ( Fig. 3g ). These findings were confirmed by quantitative real-time RT–PCR, which demonstrated increased mRNA expression of PPARγ and decreased expression of MyoD and myogenin in mutant MECs compared with control ( Fig. 3h ). Given the increased fat accumulation in muscles with altered Bmpr1a signalling, AP cells from control and Myf5 +/Cre :Bmpr1a f/f muscle were also analysed in parallel to determine possible abnormalities in this adipogenic progenitor fraction. We found that mutant AP cells displayed similar adipogenic differentiation potential to control AP cells ( Fig. 3i,j ). In addition, no decreased Bmpr1a expression was detected in mutant APs ( Fig. 3k ), as expected by the notion that intramuscular adipogenic cells derive from Myf5-negative lineage progenitors [19] , [21] , [42] . Accordingly, expression of early and mature adipocyte markers was also indistinguishable between control and mutant APs ( Fig. 3k ). Collectively, these data suggest that ablation of Bmpr1a signalling affects MECs differentiation: expression of Bmpr1a is necessary for the commitment of MECs to the myogenic lineage, while its depletion results in increased adipogenic potential of these cells. 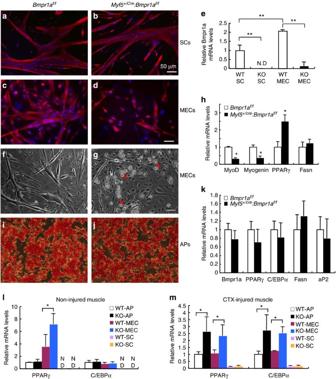Figure 3: Mutant MECs adopt an adipogenic fate. Different cell populations were separated by FACS from pooled epaxial and hypaxial muscles. (a,b) Desmin immunostaining (red) of satellite cells differentiated for 4 days in myogenic differentiation medium shows robust formation of myotubes in control and mutant cultures. (c,d) Desmin immunostaining (red) of MECs isolated fromBmpr1af/fandMyf5+/Cre:Bmpr1af/fskeletal muscle and differentiated for 4 days. Nuclei were stained with DAPI (blue). (e) Bmpr1a mRNA levels in SCs and MECs derived fromBmpr1af/f(WT) andMyf5+/Cre:Bmpr1af/f(KO) muscle. Results are shown as mean±s.d. (n=3, **P<0.01). ND, non-detectable. (f,g) MECs fromBmpr1af/fandMyf5+/Cre:Bmpr1af/fskeletal muscle differentiated in adipogenic medium. Control MECs form myotubes (f), while mutant MECs adopt an adipogenic fate (g). (h) mRNA levels for myogenic and adipogenic markers in MECs derived fromBmpr1af/fandMyf5+/Cre:Bmpr1af/fmuscle. Results are shown as mean±s.d. (n=3, *P<0.05). (i,j) Sorted AP cells fromBmpr1af/fandMyf5+/Cre:Bmpr1af/fmuscle induced to differentiate into adipocytes for 12 days before Oil Red O staining. (k) RNA isolated from cultured AP cells and analyzed for expression of Bmpr1a and adipogenic markers by real-time qRT-PCR. No differences were seen between control and mutant cells. Results are shown as mean±s.d. (n=3). (l,m) APs, SCs and MECs freshly isolated from non-injured (l) or CTX-injured muscle 4 days post-injury (m) in control and mutant mice were assayed for adipogenic marker PPARγ and C/EBPα mRNA expression by quantitative real time RT/PCR. WT:Bmpr1af/f; KO:Myf5+/Cre:Bmpr1af/f. Results are shown as mean±s.d. (n=3). Error bars indicate s.d.,n=3, *P<0.05 byt-test. Figure 3: Mutant MECs adopt an adipogenic fate. Different cell populations were separated by FACS from pooled epaxial and hypaxial muscles. ( a , b ) Desmin immunostaining (red) of satellite cells differentiated for 4 days in myogenic differentiation medium shows robust formation of myotubes in control and mutant cultures. ( c , d ) Desmin immunostaining (red) of MECs isolated from Bmpr1a f/f and Myf5 +/Cre :Bmpr1a f/f skeletal muscle and differentiated for 4 days. Nuclei were stained with DAPI (blue). ( e ) Bmpr1a mRNA levels in SCs and MECs derived from Bmpr1a f/f (WT) and Myf5 +/Cre :Bmpr1a f/f (KO) muscle. Results are shown as mean±s.d. ( n =3, ** P <0.01). ND, non-detectable. ( f , g ) MECs from Bmpr1a f/f and Myf5 +/Cre :Bmpr1a f/f skeletal muscle differentiated in adipogenic medium. Control MECs form myotubes ( f ), while mutant MECs adopt an adipogenic fate ( g ). ( h ) mRNA levels for myogenic and adipogenic markers in MECs derived from Bmpr1a f/f and Myf5 +/Cre :Bmpr1a f/f muscle. Results are shown as mean±s.d. ( n =3, * P <0.05). ( i , j ) Sorted AP cells from Bmpr1a f/f and Myf5 +/Cre :Bmpr1a f/f muscle induced to differentiate into adipocytes for 12 days before Oil Red O staining. ( k ) RNA isolated from cultured AP cells and analyzed for expression of Bmpr1a and adipogenic markers by real-time qRT-PCR. No differences were seen between control and mutant cells. Results are shown as mean±s.d. ( n =3). ( l , m ) APs, SCs and MECs freshly isolated from non-injured ( l ) or CTX-injured muscle 4 days post-injury ( m ) in control and mutant mice were assayed for adipogenic marker PPARγ and C/EBPα mRNA expression by quantitative real time RT/PCR. WT: Bmpr1a f/f ; KO: Myf5 +/Cre :Bmpr1a f/f . Results are shown as mean±s.d. ( n =3). Error bars indicate s.d., n =3, * P <0.05 by t -test. Full size image To prove that the adipogenic potential of MECs in mutant mice is not due to an adaptation to the in vitro culture conditions and that MECs with disrupted Bmpr1a signalling express adipogenic transcription factors in vivo , MECs, APs and SCs were isolated in parallel from control and Myf5 +/Cre :Bmpr1a f/f mice from uninjured or CTX-injured muscles ( Fig. 3l,m ). Freshly isolated cells were analysed by real-time PCR for expression of early (PPARγ) and mature (C/EBPα, CCAAT-enhancer-binding protein α) adipogenic markers. In MECs extracted from non-injured muscle, PPARγ expression was significantly elevated in mutant MECs compared with control MECs. Overall, PPARγ expression was higher in MECs compared with APs from either control or mutant mice ( Fig. 3l ). In contrast, satellite cells from either control or mutant mice did not express detectable levels of PPARγ or C/EBPα ( Fig. 3l ). These results demonstrate that MECs have intrinsic adipogenic potential. Following cardiotoxin injury, both PPARγ and C/EBPα expression levels were significantly elevated in MECs and APs from mutant mice compared with controls, while the level of expression in satellite cells remained very low ( Fig. 3m ). These data are in agreement with the increased adipocyte accumulation in mutant regenerating muscle, and it supports the hypothesis that both APs and MECs can contribute to adipocyte formation in regenerating muscles lacking Bmpr1a. MECs are bipotent and inhibit differentiation of adipocytes To study whether MECs gain adipogenic differentiation potential following loss of Bmpr1a expression, MECs extracted from Bmpr1a f/f muscles were treated with Cre-expressing adenovirus (Adeno Cre ) to delete the floxed Bmpr1a gene. Control Bmpr1a f/f MECs robustly differentiated into myotubes even when cultured in adipogenic medium ( Fig. 4a ), while Bmpr1a f/f MECs treated with Adeno Cre showed nearly complete inhibition of myotube formation and induction of adipocyte formation ( Fig. 4b , red arrows). Real-time RT/PCR analysis revealed that Bmpr1a expression was completely depleted in the Adeno Cre -treated cultures, accompanied by a severe reduction in MyoD and myogenin expression, while the expression of the pre-adipocyte marker PPARγ was significantly increased ( Fig. 4c ). Expression of the mature adipocyte markers Fasn and aP2, however, did not increase, suggesting that under these conditions the majority of the Adeno Cre -treated cells are immature adipocytes. To determine at the clonal level whether MECs can adopt two cell fates (myogenic or adipogenic), MECs from Bmpr1a f/f muscles were treated with or without Adeno Cre virus and individual cells from both populations were sorted into single wells of 96-well plates by FACS. Single cells were allowed to expand in growth medium for 10–12 days, followed by adipogenic differentiation. For untreated MECs, all derived clones were myogenic, which formed myotubes as determined by co-expression of desmin and MyoD ( Fig. 4d,g ). In contrast, only 20.8% of MEC clones were myogenic following Bmpr1a ablation, whereas the majority (66.7%) was adipogenic, as confirmed by expression of perilipin ( Fig. 4e,g ) or PPARγ ( Supplementary Fig. 6B ). In addition, 12.5% of Adeno Cre -treated MEC clones expressed desmin and perilipin ( Fig. 4f,g ), further supporting that MECs can adopt dual cell fate. 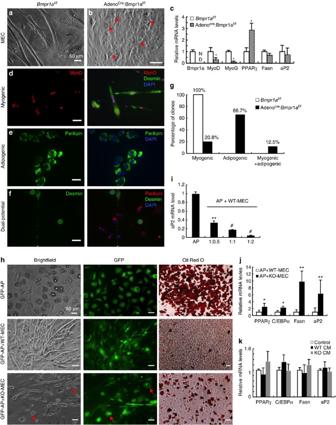Figure 4: Ablation of Bmpr1a expression in MECs results in increased adipogenesis. (a,b)Bmpr1af/fMECs treated with (b) or without (a) AdenoCrewere induced to differentiate in adipogenic medium (n=3). (a) MECs with functional Bmpr1a signalling form myotubes even when cultured in adipogenic medium. (b) MECs treated with AdenoCreexhibit decreased myotube formation and show presence of mature fat cells (red arrows). (c) Expressions of myogenic and adipogenic markers were assessed in MEC cultures treated or non-treated with AdenoCre. MyoG= myogenin. Results are shown as mean±s.d. (n=3, *=P<0.05). (d–f) Examples of myogenic (d), adipogenic (e) and dual potential (f) clones derived from four 96-well plates seeded with single untreated or AdenoCre-treated MECs assayed by immunofluorescence staining. The clonal efficiency was ~19% for untreated cells and 13% for AdenoCretreated cells, respectively. Adipogenic cells express lipid-droplet-associated protein perilipin, while myogenic cells express desmin. Scale bar, 50 μm. (g) Wild-type MECs gave rise to myogenic clones only, while MEC clones that were treated with AdenoCregave rise to mainly adipogenic clones, with significantly less myogenic clones and clones containing cells both myogenic and adipogenic. (h,i) AP cells isolated from β-actin-EGFP transgenic mice (green) were cultured alone (GFP-AP) or co-cultured with MECs derived fromBmpr1af/f(WT) orMyf5+/Cre:Bmpr1af/f(KO) muscle at the ratio of 1: 0.5, unless otherwise stated. Data are presented as mean±s.d. (n=3, **P<0.01;#P<0.001). Co-cultures were incubated in MCDB growth medium for 4 days, followed by induction of adipogenic differentiation for 9 days; red arrows indicate adipocytes. Oil red O staining was used to confirm the presence of mature adipocytes in the co-cultures. Scale bar, 50 μm. (j) Expression of early and late adipocyte markers was assessed by qRT-PCR in MEC co-cultures. Data are presented as mean±s.d. (n=3, *P<0.05; **P<0.01). (k) Adipocytes were cultured alone in control differentiation medium (control) or exposed to conditioned medium (CM) derived from WT- or KO-MEC cultures. No differences in expression of adipogenic markers were seen under these conditions, suggesting that the inhibition in AP-cell differentiation detected in the co-cultures is due to cell–cell contact between MECs and APs, rather than via inhibitory soluble factor(s). Error bars represent s.d.,n=3. Figure 4: Ablation of Bmpr1a expression in MECs results in increased adipogenesis. ( a , b ) Bmpr1a f/f MECs treated with ( b ) or without ( a ) Adeno Cre were induced to differentiate in adipogenic medium ( n =3). ( a ) MECs with functional Bmpr1a signalling form myotubes even when cultured in adipogenic medium. ( b ) MECs treated with Adeno Cre exhibit decreased myotube formation and show presence of mature fat cells (red arrows). ( c ) Expressions of myogenic and adipogenic markers were assessed in MEC cultures treated or non-treated with Adeno Cre . MyoG= myogenin. Results are shown as mean±s.d. ( n =3, *= P <0.05). ( d – f ) Examples of myogenic ( d ), adipogenic ( e ) and dual potential ( f ) clones derived from four 96-well plates seeded with single untreated or Adeno Cre -treated MECs assayed by immunofluorescence staining. The clonal efficiency was ~19% for untreated cells and 13% for Adeno Cre treated cells, respectively. Adipogenic cells express lipid-droplet-associated protein perilipin, while myogenic cells express desmin. Scale bar, 50 μm. ( g ) Wild-type MECs gave rise to myogenic clones only, while MEC clones that were treated with Adeno Cre gave rise to mainly adipogenic clones, with significantly less myogenic clones and clones containing cells both myogenic and adipogenic. ( h , i ) AP cells isolated from β-actin-EGFP transgenic mice (green) were cultured alone (GFP-AP) or co-cultured with MECs derived from Bmpr1a f/f (WT) or Myf5 +/Cre :Bmpr1a f/f (KO) muscle at the ratio of 1: 0.5, unless otherwise stated. Data are presented as mean±s.d. ( n =3, ** P <0.01; # P <0.001). Co-cultures were incubated in MCDB growth medium for 4 days, followed by induction of adipogenic differentiation for 9 days; red arrows indicate adipocytes. Oil red O staining was used to confirm the presence of mature adipocytes in the co-cultures. Scale bar, 50 μm. ( j ) Expression of early and late adipocyte markers was assessed by qRT-PCR in MEC co-cultures. Data are presented as mean±s.d. ( n =3, * P <0.05; ** P <0.01). ( k ) Adipocytes were cultured alone in control differentiation medium (control) or exposed to conditioned medium (CM) derived from WT- or KO-MEC cultures. No differences in expression of adipogenic markers were seen under these conditions, suggesting that the inhibition in AP-cell differentiation detected in the co-cultures is due to cell–cell contact between MECs and APs, rather than via inhibitory soluble factor(s). Error bars represent s.d., n =3. Full size image In addition to the evidence that MECs themselves could contribute to the fat accumulation observed in mutant mice, the possibility that interactions between MECs and APs promote intramuscular AP cells to differentiate at the expense of muscle was also examined. AP cells were isolated from β-actin-EGFP transgenic mice and cultured alone or co-seeded with different numbers of MECs from control Bmpr1a f/f mice. In contrast to the single culture of APs, adipogenic differentiation was markedly inhibited when GFP pos APs were co-cultured with WT-MECs and the degree of inhibition positively correlated with the number of MECs added ( Fig. 4h,i ). In contrast, when MECs from Myf5 +/Cre :Bmpr1a f/f mice were co-cultured with GFP pos AP cells, inhibition of adipogenic differentiation was less obvious ( Fig. 4h ) and expression of mature adipogenic markers was strongly upregulated as compared with co-culture with wild-type MECs ( Fig. 4j ). To test whether this inhibition is mediated by secreted/soluble factors, APs were cultured in conditioned medium from WT- or KO-MECs. Inhibition of adipogenesis was not observed under these conditions ( Fig. 4K ). Collectively, these studies support the conclusion that MECs with functional Bmpr1a signalling exert an inhibitory effect on adipocyte differentiation, which is likely mediated by cell–cell contact. Reduced proliferation and pSmad signalling in mutant MECs Activation of Bmpr1a signalling is mediated through phosphorylation of Smad 1, 5, 8 (Smad1/5/8) proteins [35] . To determine whether Bmp signalling was affected downstream of Bmpr1a expression in mutant mice, phospho-Smad (pSmad1/5/8) activation under basal conditions and following stimulation with Bmp4 was assessed in SCs and MECs. pSmad signalling was decreased in epaxial SCs from Myf5 +/Cre :Bmpr1a f/f mice under basal conditions and following stimulation with Bmp4, but not from MyoD +/iCre :Bmpr1a f/f mice ( Fig. 5a ). In contrast, limb SCs from either Myf5 +/Cre :Bmpr1a f/f or MyoD +/iCre :Bmpr1a f/f mice did not show any significant change in pSmad signalling ( Fig. 5b ). Accordingly, SCs from the epaxial trapezius and paraspinal muscles of Myf5 +/Cre :Bmpr1a f/f mice proliferated less efficiently than wild-type SCs, whereas SCs extracted from limb muscles were unaffected ( Fig. 5c ). SCs derived from MyoD +/iCre :Bmpr1a f/f mice exhibited either increased or similar proliferation capacity to control SCs, regardless of whether they were derived from epaxial or hypaxial (limb) muscles ( Fig. 5d ). To explain why limb SCs were not affected following Bmpr1a ablation, the expression of two additional Bmp type I receptors, Bmpr1b and activin-receptor like kinase 2 (Alk2), which could compensate for Bmpr1a decreased expression, was examined. Bmpr1b mRNA expression levels revealed a 2.6±0.8-fold increase in KO limb SCs compared with control SCs, while Alk2 expression was not changed ( Fig. 5e ). In contrast, epaxial SCs did not show compensatory upregulation of Bmpr1b or Alk2 expression ( Fig. 5f ). 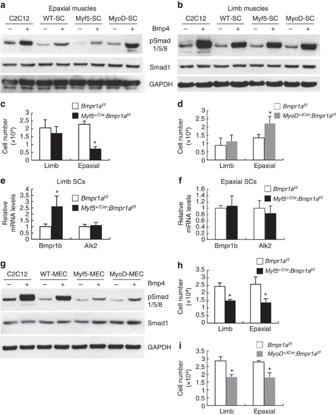Figure 5: Ablation of Bmpr1a results in decreased pSmad signalling in MECs. (a,b) Satellite cells from epaxial (paraspinal and trapezius) and limb muscles were isolated fromBmpr1af/f(WT-SC) orMyf5+/Cre:Bmpr1af/f(Myf5-SC) orMyoD+/iCre:Bmpr1af/f(MyoD-SC) mice. Cells were treated with or without 25 ng ml−1Bmp4 for 1 h, and cell lysates were analysed for activated pSmad1/5/8 expression by western blotting. C2C12 cells were treated in parallel as a positive control. Total Smad1 expression levels were similar in all samples analysed. GAPDH expression was used as a loading control. (a) Epaxial Myf5-SCs showed lower levels of activated pSmad1/5/8 under basal conditions or following stimulation with Bmp4 compared to WT-SCs. (b) In contrast, limb satellite cells from both mutant strains appeared unaffected. (c,d) Freshly isolated SCs derived from limb and epaxial muscles ofBmpr1af/forMyf5+/Cre:Bmpr1af/forMyoD+/iCre:Bmpr1af/fmice were seeded at the same cell density and the total number of live cells counted after 4 days in growth medium. No significant cell death was observed in any culture as examined by Trypan blue staining. (c) Epaxial satellite cells fromMyf5+/Cre:Bmpr1af/fmutant mice displayed decreased proliferative potential compared with control (*P<0.05), while limb satellite cells were unaffected. (d) In contrast, epaxial SCs fromMyoD+/iCre:Bmpr1af/fmice showed increased proliferative capacity compared with control, while limb SCs were again unaffected. (e,f) Relative mRNA expression of Bmpr1b and ALK2 in limbeand epaxial SCsf. Bmpr1b expression was increased in mutant limb SCs, results are shown as mean±s.d. byt-test (n=3, *P<0.05). (g) Freshly isolated MECs derived fromBmpr1af/forMyf5+/Cre:Bmpr1af/forMyoD+/iCre:Bmpr1af/fmuscles (limb and epaxial) were expanded for 4 days in growth medium and analysed in parallel for pSmad1/5/8 activation. pSmad1/5/8 activity was severely reduced in MECs from both mutant strains, both under basal conditions as well as following Bmp4 stimulation. (h,i) MECs from mutant mice displayed a reduced proliferative capacity compared with control (error bars: s.d.,n=3, *P<0.05 byt-test), regardless of whether they were isolated from epaxial or limb muscles. Figure 5: Ablation of Bmpr1a results in decreased pSmad signalling in MECs. ( a , b ) Satellite cells from epaxial (paraspinal and trapezius) and limb muscles were isolated from Bmpr1a f/f (WT-SC) or Myf5 +/Cre :Bmpr1a f/f (Myf5-SC) or MyoD +/iCre :Bmpr1a f/f (MyoD-SC) mice. Cells were treated with or without 25 ng ml −1 Bmp4 for 1 h, and cell lysates were analysed for activated pSmad1/5/8 expression by western blotting. C2C12 cells were treated in parallel as a positive control. Total Smad1 expression levels were similar in all samples analysed. GAPDH expression was used as a loading control. ( a ) Epaxial Myf5-SCs showed lower levels of activated pSmad1/5/8 under basal conditions or following stimulation with Bmp4 compared to WT-SCs. ( b ) In contrast, limb satellite cells from both mutant strains appeared unaffected. ( c , d ) Freshly isolated SCs derived from limb and epaxial muscles of Bmpr1a f/f or Myf5 +/Cre :Bmpr1a f/f or MyoD +/iCre :Bmpr1a f/f mice were seeded at the same cell density and the total number of live cells counted after 4 days in growth medium. No significant cell death was observed in any culture as examined by Trypan blue staining. ( c ) Epaxial satellite cells from Myf5 +/Cre :Bmpr1a f/f mutant mice displayed decreased proliferative potential compared with control (* P <0.05), while limb satellite cells were unaffected. ( d ) In contrast, epaxial SCs from MyoD +/iCre :Bmpr1a f/f mice showed increased proliferative capacity compared with control, while limb SCs were again unaffected. ( e , f ) Relative mRNA expression of Bmpr1b and ALK2 in limb e and epaxial SCs f . Bmpr1b expression was increased in mutant limb SCs, results are shown as mean±s.d. by t -test ( n =3, * P <0.05). ( g ) Freshly isolated MECs derived from Bmpr1a f/f or Myf5 +/Cre :Bmpr1a f/f or MyoD +/iCre :Bmpr1a f/f muscles (limb and epaxial) were expanded for 4 days in growth medium and analysed in parallel for pSmad1/5/8 activation. pSmad1/5/8 activity was severely reduced in MECs from both mutant strains, both under basal conditions as well as following Bmp4 stimulation. ( h , i ) MECs from mutant mice displayed a reduced proliferative capacity compared with control (error bars: s.d., n =3, * P <0.05 by t -test), regardless of whether they were isolated from epaxial or limb muscles. Full size image Mutant MECs from Myf5 +/Cre :Bmpr1a f/f and MyoD +/iCre :Bmpr1a f/f mice were also analysed for pSmad1/5/8 activation compared with control MECs. A significant reduction of active pSmad was seen in MECs from both Myf5 +/Cre :Bmpr1a f/f and MyoD +/iCre :Bmpr1a f/f mice under basal conditions ( Fig. 5g ). In addition, when cells were stimulated with Bmp4, pSmad1/5/8 levels increased in control C2C12 and WT MECs, but remained significantly lower in mutant cells ( Fig. 5g ). Mutant MECs from both limb and epaxial muscles also displayed substantially reduced proliferative capacity compared with control cells in both models ( Fig. 5h,i ). Collectively, these data support the conclusion that Bmpr1a signalling is important in MECs, which proliferate poorly when pSmad signalling is compromised. Moreover, epaxial SCs appear also to be affected by ablation of Bmpr1a, which may account for the reduced myofibre size in epaxial muscles of Myf5 +/Cre :Bmpr1a f/f mice. In contrast, genetic ablation of Bmpr1a in limb satellite cells is compensated by upregulation of Bmpr1b. MECs show myogenic potential in vitro and in vivo To examine the localization of MECs in vivo , muscle tissue sections were co-stained for Sca-1, CD31 and laminin, which revealed the presence of two subtypes of Sca-1 pos CD31 pos cells ( Fig. 6 ). The first one is surrounded by its own laminin staining ( Fig. 6a , arrowheads), suggesting that these cells are vascular endothelial cells. The other subtype resides interstitially between myofibres and does not have its own laminin staining ( Fig. 6b,c , arrows). Co-staining of muscle tissue sections with CD31, laminin and Pax7 indicated the presence of CD31 pos Pax7 neg cells ( Fig. 6d , arrowhead), as well as rare CD31 pos Pax7 pos cells in the interstitium ( Fig. 6e , white arrow), in addition to CD31 neg Pax7 pos satellite cells ( Fig. 6d , yellow arrow). 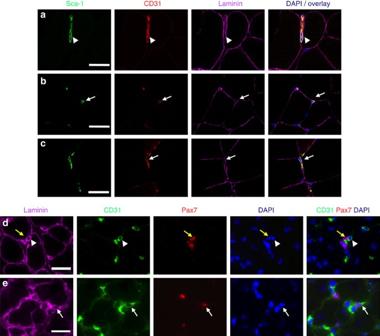Figure 6: Detection of endothelial/myo-endothelial cells (MECs) in adult mouse muscle. (a–c) Colocalization of Sca-1 (green), CD31 (red) and laminin (purple) shows co-expression of Sca-1 and CD31 in cells that reside between myofibres with (arrowheads) or without (arrows) their own basal lamina. Scale bar, 20 μm. (d,e) Immunostaining for laminin (purple) CD31 (green) Pax7 (red), and nuclei (DAPI) detects satellite cells, which reside beneath the basal lamina and are CD31negPax7pos(D, yellow arrow) as well as CD31posPax7negcells (d, white arrowheads), which constitute the vast majority of CD31poscells, as well as rare CD31posPax7poscells that reside within the interstitial space and are surrounded by laminin on both sides of the cell (e, white arrow). Scale bar, 20 μm. Figure 6: Detection of endothelial/myo-endothelial cells (MECs) in adult mouse muscle. ( a – c ) Colocalization of Sca-1 (green), CD31 (red) and laminin (purple) shows co-expression of Sca-1 and CD31 in cells that reside between myofibres with (arrowheads) or without (arrows) their own basal lamina. Scale bar, 20 μm. ( d , e ) Immunostaining for laminin (purple) CD31 (green) Pax7 (red), and nuclei (DAPI) detects satellite cells, which reside beneath the basal lamina and are CD31 neg Pax7 pos (D, yellow arrow) as well as CD31 pos Pax7 neg cells ( d , white arrowheads), which constitute the vast majority of CD31 pos cells, as well as rare CD31 pos Pax7 pos cells that reside within the interstitial space and are surrounded by laminin on both sides of the cell ( e , white arrow). Scale bar, 20 μm. Full size image To trace the developmental origin of MECs in epaxial and hypaxial muscles, Myf5- and MyoD-i Cre driver mice were crossed with reporter mice expressing yellow fluorescent protein (YFP) following Cre -mediated excision in the ROSA26 gene locus ( R26R YFP ). As expected, satellite cells from trapezius, paraspinal and limb muscles contained between 75–92% of Myf5 and MyoD-YFP expressing cells ( Supplementary Fig. 7A ). Following cytospin, expression of Pax7 was detected in >98% of the freshly isolated SCs ( Supplementary Fig. 7B ). In contrast, MECs from all muscles analysed were nearly negative for MyoD expression ( Fig. 7a , upper panels), whereas a detectable percentage of Myf5-YFP-expressing cells were seen in the MEC fraction of each muscle, particularly in the trapezius and paraspinal muscles, which contain 43±8% and 16±5% YFP pos MECs, respectively ( Fig. 7a , lower panels). Expression of Pax7 following cytospin of Myf5-positive MECs from the trapezius revealed that only ~7% of the cells expressed Pax7 on isolation ( Fig. 7b,c ), indicating that, while a substantial proportion of MECs from the trapezius are Myf5-expressing progenitors, they do not express additional myogenic markers. This is also in agreement with the finding that the majority of CD31 pos cells are Pax7 neg by immunohistochemistry. To explore whether MECs could adopt a myogenic fate following expansion in vitro , they were propagated in myogenic medium for 13 days and expression of myogenic markers was analysed. At day 3, ~97% of MECs were still positive for both Sca-1 and CD31 ( Fig. 7d ), while at day 10 and day 13 expression of CD31 was not detected ( Fig. 7d,e ). At day 10, >90% MECs were Myf5-YFP pos ( Fig. 7f ), which was also accompanied by uniform expression of Pax7 and MyoD ( Fig. 7g ). 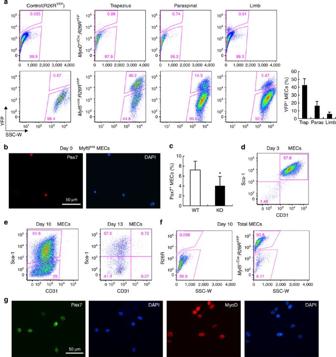Figure 7: Expression of myogenic markers in MECs following short-termin vitroculture. (a) FACS sorting plots illustrating expression of YFP in freshly isolated MECs from epaxial or hypaxial muscles ofMyoDi+/Cre:R26RYFP(top row) orMyf5+/Cre:R26RYFPreporter mice (bottom row). MyoD-YFP expression was largely negative, while Myf5-YFP expression was detected at variable percentages in all muscles, with the trapezius muscle containing the highest percentage. R26R plots are used as negative control, demonstrating no ‘leaky’ YFP expression in the studied cell populations. SSC, side scatter. Representative images are from three independent analyses. (b) Cytospins of freshly isolated Myf5posMECs fromMyf5+/Cre:R26RYFPmice stained for Pax7. Pax7 expression was detected in only ~7% MECs. (c) Pax7 staining of freshly isolated MECs fromBmpr1af/f(WT)andMyf5+/Cre: Bmpr1af/f(KO)mice revealed that KO-MECs had fewer Pax7-expressing cells than WT-MECs (n=3; *P<0.05 byt-test, error bars=s.d.). (d,e) The majority of MECs remained Sca-1posCD31posafter 3 days in culture. After 10 days, almost all MECs lost CD31 expression and a fraction became Sca-1negCD31neg. (f) After 10-day culture in myogenic medium, MECs fromMyf5+/Cre:R26RYFPmice were re-analysed for expression of Myf5-YFP, which was detected in >90% of the cells, while no YFP expression was seen in control R26R cultures. (g) Expression of Pax7 and MyoD was detected in 90±2% of MECs fromBmpr1af/fmice after 10 days in culture, confirming they were myogenic (n=3). Figure 7: Expression of myogenic markers in MECs following short-term in vitro culture. ( a ) FACS sorting plots illustrating expression of YFP in freshly isolated MECs from epaxial or hypaxial muscles of MyoDi +/Cre :R26R YFP (top row) or Myf5 +/Cre :R26R YFP reporter mice (bottom row). MyoD-YFP expression was largely negative, while Myf5-YFP expression was detected at variable percentages in all muscles, with the trapezius muscle containing the highest percentage. R26R plots are used as negative control, demonstrating no ‘leaky’ YFP expression in the studied cell populations. SSC, side scatter. Representative images are from three independent analyses. ( b ) Cytospins of freshly isolated Myf5 pos MECs from Myf5 +/Cre :R26R YFP mice stained for Pax7. Pax7 expression was detected in only ~7% MECs. ( c ) Pax7 staining of freshly isolated MECs from Bmpr1a f/f (WT) and Myf5 +/Cre : Bmpr1a f/f (KO) mice revealed that KO-MECs had fewer Pax7-expressing cells than WT-MECs ( n =3; * P <0.05 by t -test, error bars=s.d.). ( d , e ) The majority of MECs remained Sca-1 pos CD31 pos after 3 days in culture. After 10 days, almost all MECs lost CD31 expression and a fraction became Sca-1 neg CD31 neg . ( f ) After 10-day culture in myogenic medium, MECs from Myf5 +/Cre :R26R YFP mice were re-analysed for expression of Myf5-YFP, which was detected in >90% of the cells, while no YFP expression was seen in control R26R cultures. ( g ) Expression of Pax7 and MyoD was detected in 90±2% of MECs from Bmpr1a f/f mice after 10 days in culture, confirming they were myogenic ( n =3). Full size image The in vivo myogenic potential of cultured MECs was assessed by injecting 5 × 10 4 MECs isolated from β-actin-EGFP transgenic mice into the TA muscles of C57BL6 recipient mice ( Fig. 8a ). In parallel, satellite cells were isolated and injected as a positive control for successful engraftment. One month following intramuscular injection of SCs or MECs into TA muscles, transplanted mice displayed obvious presence of GFP-expressing myofibres, demonstrating in vivo myogenic differentiation capacity for MECs ( Fig. 8b,c ). Thus, while the majority of MECs do not express Pax7 or MyoD on isolation, they acquire expression of myogenic markers following culture in vitro and fuse to myofibres in vivo . 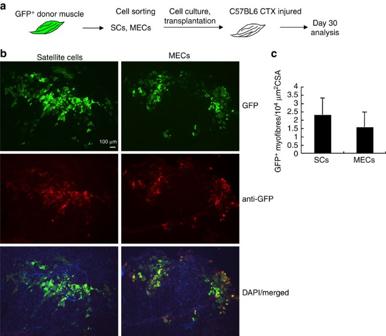Figure 8: MECs can engraft and fuse into myofibres following intramuscular transplantation. (a) Schematic representation of intramuscular transplantation of SCs and MECs. (b) Detection of GFP-positive myofibres from C57BL6 TA muscles transplanted with GFPposSCs or MECs (n=4/group). The specificity of GFP-positive myofibres was confirmed by immunostaining with an anti-GFP antibody. (c) MECs showed robust and comparable engraftment as SCsin vivo(n=4; error bars=s.d.). Figure 8: MECs can engraft and fuse into myofibres following intramuscular transplantation. ( a ) Schematic representation of intramuscular transplantation of SCs and MECs. ( b ) Detection of GFP-positive myofibres from C57BL6 TA muscles transplanted with GFP pos SCs or MECs ( n =4/group). The specificity of GFP-positive myofibres was confirmed by immunostaining with an anti-GFP antibody. ( c ) MECs showed robust and comparable engraftment as SCs in vivo ( n =4; error bars=s.d.). Full size image VE-cadherin pos cells do not significantly contribute to muscle To address whether MECs can contribute to developing or regenerating muscle in vivo , tracing using a marker expressed by MECs but absent in SCs or APs was performed. Since CD31 Cre mice are not available, we utilized VE-cadherin, a marker expressed in nearly all MECs by antibody analysis, whereas APs and SCs were negative ( Fig. 9a ). Tracing of MECs in developing muscle was tested using a VE-cadherin Cre (Cdh5 Cre ) driver [43] crossed with a R26R YFP reporter mouse. Analysis of Cdh5 Cre :R26R YFP mice showed that approximately half of the MECs (43–57%) were YFP positive under these conditions and therefore traceable ( Fig. 9b ). The VE-cadherin Cre driver mice were also crossed with R26 NZG reporters, which resulted in Cre-dependent nuclear LacZ gene expression [44] . Analysis of tissue sections from the trapezius showed that the vast majority of nuclear LacZ-expressing cells did not incorporate into myofibres and were located interstitially between myofibres ( Fig. 9c–g , black arrows), consistent with findings reported by other laboratories on limb muscles [17] , [23] . β-Galactosidase (β-gal)-positive nuclei within myofibres were also noted ( Fig. 9c–g , red arrows), but these were at very low levels (<1% of myonuclei). Co-staining of X-gal and laminin confirmed the presence of β-gal-positive myonuclei underneath the basal lamina ( Fig. 9h , red arrows). Cardiotoxin injury was also performed in these mice and regenerating muscles were harvested 23 days following injury and stained for β-gal. Again, the majority of β-gal-expressing cells were located in the interstitium ( Fig. 9i–k , black arrows), although β-gal-expressing centrally located nuclei were again noted at very low levels ( Fig. 9i–k , red arrows). Thus, Cdh5 -expressing cells do not contribute to developing or regenerating muscle at biologically significant levels. 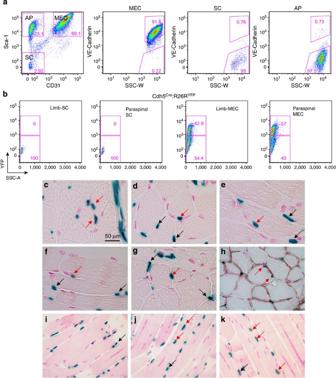Figure 9: Modest contribution of MECs to developing muscle via Cdh5Crelineage tracing. (a) FACS analysis of VE-cadherin expression on MECs, SCs and APs via antibody staining. MECs were nearly all positive for VE-Cadherin, while the vast majority of SCs and APs were negative. (b) Detection of VE-cadherin-YFP expression in SCs and MECs using Cdh5Cre:R26RYFPmice. Again, SCs were all negative for VE-cadherin expression, while only ~40–50% of MECs were viewed as YFP positive, demonstrating an overall lower labelling yield of MECs when compared with the antibody staining. (c–g) Detection of β-gal-positive nuclei (blue) in tissue sections of trapezius muscles of Cdh5Cre:R26NZGmice. While most β-gal-positive nuclei were located between myofibres (black arrows), a very small proportion was also seen incorporated into myofibres (red arrows), as also documented by laminin co-staining (h, brown). (i–k) The same results were obtained for CTX-injured TA muscle. Figure 9: Modest contribution of MECs to developing muscle via Cdh5 Cre lineage tracing. ( a ) FACS analysis of VE-cadherin expression on MECs, SCs and APs via antibody staining. MECs were nearly all positive for VE-Cadherin, while the vast majority of SCs and APs were negative. ( b ) Detection of VE-cadherin-YFP expression in SCs and MECs using Cdh5 Cre :R26R YFP mice. Again, SCs were all negative for VE-cadherin expression, while only ~40–50% of MECs were viewed as YFP positive, demonstrating an overall lower labelling yield of MECs when compared with the antibody staining. ( c – g ) Detection of β-gal-positive nuclei (blue) in tissue sections of trapezius muscles of Cdh5 Cre :R26 NZG mice. While most β-gal-positive nuclei were located between myofibres (black arrows), a very small proportion was also seen incorporated into myofibres (red arrows), as also documented by laminin co-staining ( h , brown). ( i – k ) The same results were obtained for CTX-injured TA muscle. Full size image Satellite cells are the tissue-specific stem cells of skeletal muscle [45] , [46] , [47] . Additional progenitors located interstitially between myofibres are also present and these consist of various subgroups of cells [12] , [39] , [40] , [48] whose developmental origin and function have not been fully elucidated. Even less defined are the signalling mechanisms that might influence the fate of these progenitors towards a specific cell lineage. Bone morphogenetic protein signalling regulates the development and differentiation of a variety of tissues [49] , [50] , [51] , [52] , [53] . In developing skeletal muscle, Bmp signalling inhibits myogenic differentiation and controls the number of fetal muscle progenitors and satellite cells [54] , [55] , [56] . Postnatally, inhibition of Bmp signalling induced by short-term RNAi induced premature differentiation of satellite cells [57] . TGFβ and Bmp signalling also control the overall muscle mass through myofibres growth, which is mediated via multiple downstream signalling pathways [33] , [34] . Our previous studies in human fetal muscle identified Bmp4 and Bmpr1a as a ligand-receptor signalling mechanism between mononuclear cells, through which expansion of interstitial progenitors occurred [24] . Secretion of Bmp4 from side population cells triggered the expansion of interstitial cells co-expressing Myf5 and Bmpr1a [24] . However, neither whether these Myf5 pos Bmpr1a pos cells are developmentally bona fide myogenic progenitors, nor the exact function of Bmp signalling in these progenitors could be addressed using human samples. In the present study, we generated conditional mouse models that ablated Bmpr1a expression specifically in Myf5- or MyoD-expressing progenitors to investigate how loss of Bmpr1a signalling impacts either satellite cells, or intramuscular interstitial progenitors, or both of these cell groups. Overall, Myf5 +/Cre :Bmpr1a f/f mice displayed a more severe phenotype than MyoD +/iCre :Bmpr1a f/f mice, suggesting that Myf5-expressing cells distinct from MyoD pos satellite cells are implicated. Indeed, the progenitors implicated (MECs) are Sca-1 pos CD31 pos CD45 neg and PDGFRα neg by cell surface markers and are also MyoD neg . MECs can adopt a myogenic specification following culture in vitro and intramuscular transplantation in vivo , although the contribution of MECs to developing and regenerating muscles is very limited based on VE-cadherin tracing. Thus, the primary function of these cells in vivo is likely not to contribute to muscle formation, but to support satellite cell activity in inhibiting the differentiation of intramuscular adipogenic progenitors. MECs require expression of Bmpr1a to reveal their myogenic potential. Indeed, wild-type MECs differentiated into myotubes both in bulk cultures as well as when grown as clones even under conditions that favour adipogenic differentiation. In contrast, ablation of Bmpr1a in MECs resulted in severely reduced myogenic activity and increased differentiation into adipocytes. More recently, satellite cells have been shown to adopt a brown adipocyte fate when microRNA-133 expression is downregulated [58] . This appears to be an independent mechanism of cell fate-conversion, as in the current study satellite cells lacking Bmpr1a remained myogenic even when cultured in adipogenic differentiation medium for 12 days. The development of limb satellite cells in a Bmpr1a-flawed environment did not seem to affect their activity, possibly because of the activation of compensatory mechanisms, such as the increased expression of the alternative receptor Bmpr1b. However, normal limb satellite cell activity was not sufficient to prevent abnormal intramuscular adipogenesis, pointing to a function of MECs in regulating the proliferation and/or differentiation of adipocytes. Altogether, these findings indicate that Bmpr1a signalling in MECs may block MECs themselves from adopting an adipogenic fate, as well as inhibiting the activity of endogenous intramuscular adipocyte progenitors, as demonstrated by our clonal and in vitro co-culture studies. In addition to fat infiltration, mutant Myf5 +/Cre :Bmpr1a f/f mice exhibited smaller epaxial muscles than wild-type littermates. This phenotype is likely due to impaired function of both satellite cells and interstitial MECs, as reduced SC proliferation and pSmad signalling was also seen in affected epaxial muscles. Collectively, these studies suggest that both SCs and MECs function contribute to the proper formation of epaxial muscles and that Bmpr1a signalling is critical for the proliferation of both cells types. While ablation of Bmpr1a in epaxial muscles using a Myf5 driver influenced the overall size and number of myofibres, limb satellite cells where Bmpr1a expression was ablated using a MyoD-iCre driver did not seem affected, nor were the size or number of myofibres of the limb muscles analyzed. These results support the conclusion that intramuscular Myf5-expressing cells that are not satellite cells are most affected by altered Bmpr1a signalling. In support of these findings, recent studies in the extraocular muscle (EOM) highlighted the existence of ancestral Myf5-expressing progenitors that do not express MyoD and exhibit fibro-adipogenic potential. These cells might be derived from the neural crest, as they might be related to cells of Pax-3 origin [59] . While ancestral expression of Pax3 was not assessed in MECs, nor Bmpr1a expression was tested in this EOM cell fraction, future studies should address similarities between these cell fractions and a possible common developmental origin. Even though several cell surface and intracellular markers were used to define MECs in the present study, most of these markers are expressed in more than one cell type in skeletal muscle, particularly in cells that are not sublaminar (non-satellite cells) and reside between myofibres or near the vasculature. Therefore, the identification of additional markers unique to some of these interstitial cell fractions, which will distinguish them from one another, is one of the present challenges that need to be overcome to provide better tools to study these different subclasses of interstitial cells. Tissue localization of MECs in uninjured and regenerating muscle revealed the presence of rare intermyofibre mononuclear cells that were surrounded by laminin staining in both the cytoplasmic and extracellular sides and expressed Pax7. These rare intermyofibre Pax7-expressing cells might be a derivative of satellite cells that have separated from myofibres, as previously described for ageing muscle or following denervation [60] , [61] , or, alternatively, it might be a distinct cell type. In Pax7-ZsGreen reporter mice, 3–16% of Pax7-expressing cells are also positive for Sca-1 (ref. 62 ), a marker used in conjunction with CD31 to exclude interstitial cells in routine methods that purify satellite cells [19] , [63] , [64] . Thus, these Sca-1 + Pax7-ZsGreen cells might include the interstitial Pax7-positive cells localized in the present study. The majority of MECs are not Pax7-positive in vivo , but they gain Pax7, Myf5 and MyoD expression when cultured in vitro . This feature is similar to interstitial cells expressing PW1 that have been described in skeletal muscle as a potential stem cell fraction that participates in myogenesis [16] . Both PW1 + cells and MECs express Sca-1, but PW1 cells do not express CD31 by immunohistochemistry [16] and MECs exhibit very low expression of PW1 by real-time RT/PCR, suggesting low or minimal overlap between PW1 + cells and MECs. Expression of NG2 was also nearly undetectable in MECs, supporting low or minimal overlap between MECs and pericytes [17] . Sca-1 expression has been generally associated with non-satellite cell fractions in skeletal muscle [19] , [63] , [64] , although it has been complicated by the transient nature of Sca-1 expression associated with the muscle microenvironment, which influences the proliferation and differentiation of myogenic progenitors [65] , [66] . Thus, additional prospective markers that unequivocally distinguish satellite cells from other interstitial progenitors with myogenic potential will provide potentially better tools to distinguish these cell types, although it cannot be excluded that these distinctions might be blurred or made difficult by intrinsic heterogeneity within the cell fractions or by the possibility that a common progenitor might give rise to both. In summary, the present study demonstrates that genetic disruption of Bmpr1a signalling in skeletal muscle suppresses MECs proliferation and yields to increased intramuscular fat. The abnormal fat accumulation observed in mutant muscle might be due to a dual effect: an increased adipogenic differentiation potential of MECs, which could be bipotent progenitors (muscle and fat) and a decreased inhibitory role of SCs and MECs on adipogenic progenitors. Thus, interstitial myo-endothelial progenitors might modulate the balance between muscle and fat, and this function is dependent on Bmp signalling. Ectopic fat cell accumulation is often seen in diseased or ageing muscle. The current findings may highlight a pathway through which inhibition of adipogenic formation could be targeted in these conditions. Animals Myf5 +/Cre (ref. 26 ) and MyoD +/iCre mice [29] were kindly provided by Dr Amy Wagers (Joslin Diabetes Center, MA) and Dr David Goldhamer (University of Connecticut, CT), respectively. Cdh5 Cre (VE-cadherin Cre stock 006137), Rosa26 YFP , R26 NZG and C57BL/6-Tg(ACTBEGFP) 1Osb/J (β-actin-EGFP) mice were obtained from the Jackson Laboratory. Bmpr1a f/f mice [25] were crossed with Myf5 +/Cre or MyoD +/iCre mice to generate mice with muscle lineage-specific deletion of Bmpr1a ( Myf5 +/Cre :Bmpr1a f/f or MyoD +/iCre :Bmpr1a f/f ). Muscles from both male and female mice of age 4 to 10 weeks were used for FACS analysis. Animals were housed and handled in accordance with the guidelines of the Boston Children’s Hospital subcommittee for animal research. All experimental procedures were performed as described in a protocol approved by the IACUC at Boston Children’s Hospital. Cardiotoxin injury Muscle injury was induced by injection of cardiotoxin (15 μl of 0.5 μg μl −1 stock) from Naja mossambica (Sigma-Aldrich, MO) into the TA or GA muscle of adult Bmpr1a f/f , Myf5 +/Cre :Bmpr1a f/f or MyoD +/iCre :Bmpr1a f/f mice. Muscles were harvested at various time points after injection for histological, RNA and protein analyses. Contralateral, uninjected TA or GA muscles were used as controls. Histology and Immunofluorescence Mice were killed by CO 2 inhalation. For cross-sections of the paraspinal area, the skin was peeled off, and the chest and abdomen were cut open. The whole body was immersed in Bouin’s fixative solution, and the samples were processed by the Rodent Histopathology Core Facility at Harvard Medical School. Cross-sections of the paraspinal area were obtained for the determination of myofibre size and the number of myofibres. For trapezius, non-injured or CTX-injured TA and GA muscles were dissected, embedded for cryostat sectioning and rapidly frozen in cold isopentane [67] . Muscle tissue sections (10 μm) were subjected to H&E staining and the myofibre size was determined by measuring the cross-sectional area (CSA). Regeneration was analysed by measuring the diameter of regenerating myofibres with centrally localized nuclei. Measurements were performed using Image J software (National Institute of Health; http://rsb.info.nih.gov/ij/ ). For immunofluorescence, cells or tissue sections were fixed in 4% paraformaldehyde for 10 min, permeabilized with 0.1% Triton X-100 in PBS for 10 min and blocked with 1% BSA and 5% donkey serum in PBS for 1 h. Cells or tissue sections were incubated with the primary antibodies overnight at 4 °C diluted as follows: rabbit anti MyoD (Santa Cruz Biotech, 1:50), mouse anti-desmin (DAKO, 1:100), biotin anti-mouse Sca-1 (Biolegend, 1:100), rat anti- mouse CD31 (BD Pharmingen, 1:100), rabbit anti-laminin (Sigma-Aldrich, 1:500), rabbit anti-perilipin (Sigma-Aldrich, 1:150). Slides were washed in 1 × PBS three times, 10 min each and incubated with the appropriate secondary antibodies for 1 h at room temperature. Slides were washed again with PBS as above and mounted in Vectashield (Vector Laboratories, CA) supplemented with 100 ng ml −1 DAPI to visualize nuclei. Epifluorescent images were captured using a Nikon Eclipse E-1000 microscope equipped with a Hamamatsu digital camera, and images were acquired using Openlab software version 3.1.5 (Improvision). Pax7 immunofluorescence on tissue sections Muscle tissue sections (10 μm) were prepared using a cryostat and let dry at room temperature (RT). Sections were fixed in 2% PFA diluted in PBS for 10 min, then washed 3 × 5 min in PBS. Sections were dehydrated with gentle shaking in 50, 70, 80, 95 and 100% (twice) ethanol/water. Slides were incubated in xylene 2 × 3 min and rehydrated (3 min each, gentle shaking) in 95 and 70% ethanol, followed by 1 × PBS. To unmask antigens, slides were incubated for 20 min in 0.01 M NaCitrate pH 6.0 in a steamer, then rinsed with 1 × PBS. Slides were then permeabilized with 0.5% triton X -100 in PBS for 10 min, then rinsed with 1 × PBS. Sections were blocked in blocking solution (2% horse serum, 2% goat serum 2% BSA (fraction V) 0.1% triton X 100, made in PBS) for 30 min at RT, followed by blocking with MOM kit blocking solution (Vector labs) for 30 min at RT. Primary antibodies were diluted in MOM diluent and incubated overnight at 4°C as follows: mouse anti-Pax7 (Developmental Studies Hybridoma Bank, concentrated supernatant, diluted 1:100), rabbit anti-laminin (Sigma-Aldrich, 1:500). Sections were rinsed with PBS (4 × 5 min each), then appropriate secondary Abs (Jackson ImmunoResearch) were diluted in MOM diluent (1:100) and incubated for 1 h at RT. Slides were then washed for 4 × 5 min in PBS and mounted in DAPI/Vectashield mounting medium. Slides were analysed and images acquired as described above. X-gal Staining Muscle tissues were excised and frozen in liquid nitrogen-cooled isopentane. Tissue sections (10 μm) were fixed in 0.2% glutaraldehyde, 2 mM MgCl 2 for 10 min at room temperature and then washed briefly two times in PBS and one time with LacZ wash buffer containing 2 mM MgCl 2 , 0.01% Deoxycholate, 0.02%NP-40 in PBS. Fixed sections were stained overnight in 5-bromo-4-chloro-3-indolyl-‘-D-galactopyranoside (X-gal) working solution at 37 °C. The X-gal working solution contained 5 mM potassium hexacyanoferrate (III), 5 mM potassium hexacyanoferrate (II) trihydrate and 1 mg ml −1 of X-gal in Lacz wash buffer. Following the overnight incubation, sections were washed three times for 10 min per wash in PBS, stained with nuclear fast red for 3 min, dehydrated in 70, 95 and 100% ethanol for 2 min each, cleared for 1 min in xylene and then mounted on a coverslip using Permount mounting media. For co-staining of X-gal and laminin, tissue sections were stained with the laminin antibody as described above and HRP-conjugated anti-rabbit secondary antibody, followed by 3,3′-diaminobenzidine (DAB) detection (Vector labs). Afterwards, the specimens were stained for X-gal. Oil Red O staining Lipid accumulation was visualized by staining cells or tissue sections with the lipid-specific dye Oil Red O (Sigma-Aldrich, MO). In brief, 8–10 μm tissue sections or cells were fixed with 10% formalin and rinsed with tap water for 1–10 min before being rinsed in 60% isopropanol. Slides were then placed in 0.25% Oil Red O solution in isopropanol for 8–10 min in a 60 °C oven. Slides were rinsed again in 60% isopropanol, and nuclei were stained in alum haematoxylin for 1 min, followed by a rinse in distilled water and mounted in aqueous solution. Fluorescence-activated cell sorting Pooled epaxial and hypaxial skeletal muscles were harvested, minced using sterile scalpels and digested at 37 °C for 45 min using a final concentration of 1.2 U dispase II (Roche Applied Science, IN) and 5 mg collagenase D (Roche Applied Science, IN) per gram of tissue with gentle trituration every 15 min. Digestion was terminated by addition of growth medium. Digested samples were filtered through a 40-μm cell strainer, spun down and treated with RBC lysis buffer (Qiagen, Valencia, CA). Cells were spun down and resuspended in ice-cold 1 × HBSS (Hank’s buffered salt solution, Invitrogen) containing 0.5% BSA at a concentration of 2 × 10 7 cells ml −1 . Antibodies were added at the following dilutions: anti-mouse CD45 (1:300, PE-Cy7 conjugate, clone 30-F11), anti-mouse Sca-1 (Ly-6A/E, 1:100, FITC or APC-Cy7 conjugate, clone E13-161.7), anti-mouse CD31 (1:200, APC or PE conjugate, clone MEC13.3) (all from BD Pharmingen, CA), anti-mouse PDGFR1α (1:100, APC or biotin conjugate, clone APA5, Biolegend, CA), anti-mouse CD106 (VCAM-1, 1:75, FITC or PE conjugate, clone 429, Biolegend, CA, anti-mouse VE-cadherin (1:100, clone 11D4.1, BD Pharmingen, CA). Cells and diluted antibodies were incubated on ice for 20 min, washed with cold 1 × HBSS/ 0.5%BSA and resuspended at a concentration of 10 7 cells ml −1 . To select for live cells by flow cytometry, calcein blue (Invitrogen, CA) was added at a final concentration of 4.65 μg ml −1 , and propidium iodide (PI, Sigma-Aldrich, MO) was added at a final concentration of 1 μg ml −1 . Live cells were selected by positive staining for calcein blue and negative staining for PI. Cells were sorted on either a FACSVantage SE or BD FACSAria flow cytometer (both from Becton Dickinson, NJ). FACS data were collected using CellQuest software version 3.3 or DIVA software (Becton Dickinson) and analysed using Flowjo software (Tree Star, Macintosh version 6.4.7). In vitro primary cell culture Satellite cells were plated on tissue culture dishes coated with Matrigel (BD Bioscience, MA) and cultured in growth medium (1:1 mixture of DMEM-high glucose and Ham’s F-10 medium; 20% fetal bovine serum, 5 ng ml −1 basic fibroblast growth factor, 100 U ml −1 penicillin, 100 μg ml −1 streptomycin and 2 mM L -glutamate). Myoblast differentiation was induced by switching cells from growth to differentiation medium (DMEM with low glucose, 2% horse serum, 100 U ml −1 penicillin, 100 μg ml −1 streptomycin and 2 mM L -glutamate). Cells were differentiated for 4 days under these conditions and monitored for myotube formation. To expand MECs and APs, freshly isolated cells were propagated in MCDB medium containing 60% DMEM with low glucose (Invitrogen, CA) and 40% MCDB201 (Sigma-Aldrich, MO), supplemented with 100 U ml −1 penicillin and 100 μg ml −1 streptomycin (Invitrogen, CA). The medium was supplemented with 2% FBS, 1 × insulin-transferrin-selenium mix, 1 × linoleic acid conjugated to BSA, 1 nM dexamethasone and 0.1 mM L-ascorbic acid 2-phosphate (all from Sigma-Aldrich, MO). The following growth factors were also added to the medium: 10 ng ml −1 epidermal growth factor (PeproTech, NJ), 10 ng ml −1 leukemia inhibitory factor (Millipore, MA), 10 ng ml −1 platelet-derived growth factor BB (PeproTech, NJ) and 5 ng ml −1 basic fibroblast growth factor (Sigma-Aldrich, MO) [42] . To assay for proliferation, freshly isolated SCs and MECs were plated at 2,500 cells per well and 5,000 cells per well, respectively, in 24-well plates, and the total number of live cells was counted 4 days after culture in growth medium. Dead cells were stained by Trypan blue but were found not to be different in number between cultures. To induce adipogenic differentiation, cells were treated for 48 h with MCDB medium containing 5 μg ml −1 human insulin (Roche Applied Science, IN), 50 μM indomethacin, 1 μM dexamethasone, 0.5 μM isobutylmethylxanthine (IBMX) and 1 nM 3, 3′, 5-triiodo- L -thyronine (T3) (all from Sigma-Aldrich, MO), followed by further differentiation for 7 days in MCDB medium with the addition of T3 and insulin only. Adeno Cre virus (Gene Transfer Vector Core, University of Iowa, Iowa) was applied at a concentration of 50 p.f.u. per cell. For co-culture, 5 × 10 4 AP cells sorted from β-actin-EGFP transgenic mice and 2.5 × 10 4 MECs derived from Bmpr1a f/f or Myf5 +/Cre :Bmpr1a f/f muscle were co-seeded in each well and cultured in MCDB growth medium for 4 days followed by adipogenic differentiation for 9 days. For conditioned cultures, MECs from Bmpr1a f/f or Myf5 +/Cre :Bmpr1a f/f muscle were expanded in MCDB growth medium for 4 days and were then treated with adipogenic medium for 9 days. The supernatant was collected every other day, filtered through a 0.45-μm filter and used as conditioned medium (mixed with fresh medium in a 1:1 ratio) in the cultures containing GFP pos AP cells. Clonal assay MECs isolated from Bmpr1a f/f muscles were treated with or without Adeno Cre virus at a concentration of 50 p.f.u. per cell for 48 h. Single cells were then sorted to 96-well plate by FACS and cultured with conditioned medium (MCDB growth medium collected from MEC proliferating culture, filtered and mixed with fresh medium in a 1:1 ratio) until colony formed. Four 96-well plates were generated for control cells and for cells treated with Adeno-Cre. Clones were then induced for adipogenic differentiation as described above. Western blot analyses Protein lysates were obtained from freshly isolated or cultured cells. Cells were lysed on ice for 15 min in 0.2 ml lysis buffer (50 mM Tris, pH 7.4, 150 mM NaCl, 1% NP-40, 0.1% SDS and Halt Protease Inhibitor Cocktail (Pierce Biotechnology). Cell lysates were collected and centrifuged at 15,000 g for 10 min at 4 °C. Protein concentration was determined using the BioRad Bradford assay. Protein lysates were analysed on Invitrogen NuPage Novex Bis-Tris 4–12% gradient gels with MES-SDS buffer. Gels were transferred onto nitrocellulose using the Invitrogen NuPage Transfer system. Western blots were performed using antibodies recognizing pSmad 1/5/8, pSmad2, Smad1 (Cell Signaling Technology, MA), Pax7 (Developmental Studies Hybridoma Bank, concentrated supernatant) and glyceraldehyde 3-phosphate dehydrogenase (GAPDH) (Santa Cruz Biotechnology, CA), all diluted 1:1,000. RNA isolation and Quantitative RT-PCR analysis Total RNA was isolated from tissues or cultured cells using Tri-reagent (Molecular Research Center, OH). Reverse transcription was performed using the Invitrogen Superscript III First Strand Synthesis kit for RT–PCR according to the manufacturer’s instructions (Invitrogen, CA), starting with 1 μg of total RNA. Primers were added at a final concentration of 80 nM, and the sequences are listed in Supplementary Table 1 . Quantitative real-time PCR was performed with the SYBR Green PCR master mix kit (Applied Biosystems, CA) using an ABI7900HT PCR machine under ‘default’ conditions: 50 °C for 2 min and 95 °C for 10 min, followed by 40 cycles of amplification at 94 °C for 15 s and 60 °C for 1 min. Melting curves for each primer pair were assessed to ensure specific amplification. The transcript levels were normalized to those of GAPDH. In vivo transplantation of MECs and SCs MECs and SCs sorted from β-actin-EGFP transgenic skeletal muscle were expanded for 5 days in culture and then 50,000 cells were transplanted into the TA muscle of C57BL6 mice. The TA muscle was subjected to cardiotoxin injury 1 day before cell transplantation. After 30 days, the recipient muscle was analysed for GFP-positive myofibres as previously described [68] . Statistical analysis All values are presented as the mean±s.d. from at least three independent experiments unless otherwise stated. Two-tailed Student’s t -test and one-way ANOVA were employed for statistical analyses with two groups and more than two groups, respectively. P -values less than 0.05 were considered to represent statistically significant differences. How to cite this article: Huang, P. et al . Intramuscular adipogenesis is inhibited by myo-endothelial progenitors with functioning Bmpr1a signalling. Nat. Commun. 5:4063 doi: 10.1038/ncomms5063 (2014).